Continent-wide panmixia of an African fruit bat facilitates transmission of potentially zoonotic viruses The straw-coloured fruit bat, Eidolon helvum , is Africa’s most widely distributed and commonly hunted fruit bat, often living in close proximity to human populations. This species has been identified as a reservoir of potentially zoonotic viruses, but uncertainties remain regarding viral transmission dynamics and mechanisms of persistence. Here we combine genetic and serological analyses of populations across Africa, to determine the extent of epidemiological connectivity among E. helvum populations. Multiple markers reveal panmixia across the continental range, at a greater geographical scale than previously recorded for any other mammal, whereas populations on remote islands were genetically distinct. Multiple serological assays reveal antibodies to henipaviruses and Lagos bat virus in all locations, including small isolated island populations, indicating that factors other than population size and connectivity may be responsible for viral persistence. Our findings have potentially important public health implications, and highlight a need to avoid disturbances that may precipitate viral spillover. Recent studies have demonstrated the potential of bats to act as reservoirs of zoonotic pathogens (as reviewed in Hayman et al. [1] ). One example is the common and conspicuous straw-coloured fruit bat ( Eidolon helvum ), which has been identified as a reservoir host for Lagos bat virus (LBV, family Rhabdoviridae, genus Lyssavirus ) [2] and henipaviruses (family Paramyxoviridae) [3] in mainland Africa. E. helvum is a gregarious, predominantly tree-roosting species and large roosts (sometimes numbering more than one million bats) frequently exist in close proximity to large human settlements, including Accra (Ghana), Abidjan (Côte d'Ivoire), Dar es Salaam (Tanzania), Lagos (Nigeria) and Kampala (Uganda) [4] . Much of the serological evidence for zoonotic pathogens in bats comes from single cross-sectional studies, with few conducted longitudinally or across a representative proportion of the entire species range. However, longitudinal surveys of E. helvum colonies in Ghana have demonstrated relatively high roost-level seroprevalences to LBV over multiple years, which increase with bat age [5] . These findings indicate endemic circulation with horizontal transmission, making E. helvum a true reservoir host of LBV in that country. Moreover, neutralizing antibodies to LBV have also been detected in cross-sectional serological surveys in Kenya [6] and Nigeria [7] and LBV has been isolated from a small number of sick or dead wild E. helvum bats in Nigeria, Senegal and Kenya (as reviewed in Banyard et al. [2] ). Old World fruit bats (Pteropodidae) are the principal reservoir hosts of henipaviruses [8] , with flying fox populations ( Pteropus spp.) found to harbour Nipah virus (NiV) in Southeast Asia, and both Hendra virus (HeV) and Cedar virus (CedPV) in Australia. NiV and HeV are highly pathogenic in humans and other mammals, yet the recently discovered CedPV differs in its apparent apathogenicity in laboratory animal species [9] . Cross-neutralizing antibodies to HeV and NiV have been detected in sympatric Pteropus spp. and Madagascan fruit bats ( E. dupreanum) [10] , and Hayman et al. [3] first documented antibodies to henipaviruses in bats outside the range of Pteropus spp, with a 40% seroprevalence being found in E. helvum in Ghana. These serological findings were recently supported by the detection of henipavirus-like RNA in E. helvum in Ghana and central Africa [11] , [12] , [13] ; yet, although a full genome sequence for one of these African henipavirus-like viruses was obtained [13] , live viruses have not yet been isolated. These findings collectively highlight the potential for zoonotic pathogen spillover from E. helvum to humans, with routes of infection being via urine [12] , faeces [13] or the hunting and preparation of bat meat for food [14] . However, no such spillovers have been reported for LBV or African henipaviruses. This might be because spillover has not yet occurred, or it might reflect poor medical surveillance capabilities in much of Africa, and the lack of availability of specific diagnostic assays [15] . Much is yet to be understood regarding the host response to natural lyssavirus and henipavirus infections in bats; experimental inoculations have yielded inconsistent results across individuals and studies. Bats infected with lyssaviruses may or may not develop clinical signs corresponding to those seen in other mammals (as reviewed in Banyard et al. [2] ), whereas no clinical illness has been observed in bats infected with henipaviruses [8] . Acute antibody responses have been observed for both viruses after experimental infection, with boosted titres upon reinfection [8] , [16] . An assumption could follow that these infections are immunizing in bats, however, seroconversion is not universally observed, and therefore this remains open to challenge. Typically, pathogens causing acute immunizing infections require large host population sizes and a ‘critical community size’ (CCS) for persistence is expected unless birth rates are very high. Many uncertainties also remain regarding the specific viral transmission dynamics in E. helvum . Key aspects of this species’ ecology might further increase potential for viral persistence within populations. In particular, it is a migratory species that comprises both permanent and seasonal colonies across much of sub-Saharan Africa [4] and a small number of offshore islands, including those in the Gulf of Guinea [17] ( Fig. 1 ). However, the widespread and continuous distribution represented in Fig. 1 over-simplifies a more intricate distribution pattern, comprising aggregated populations across a connected, rather than continuous, landscape [18] . Annual seasonal migrations result in abrupt fluctuations in the size of permanent colonies, and also in the formation of solely seasonal colonies. For example, the largest known E. helvum colony in Kasanka National Park in Central Zambia is populated rapidly each year to reach an estimated 1.5 million individuals [19] , and persists for just 2 ½ months. Satellite telemetry studies indicate that these bats are capable of migrating vast distances (for example, up to 370 km in one night and ~2,500 km over 5 months) [20] . It has been suggested that migration occurs along a ‘north–south’ axis, with seasonal movements following latitudinal shifts of the Intertropical Convergence Zone weather system [20] , [21] ; however, the routes and drivers of migrations are not fully understood. Such large-scale movements are expected to lead to widespread gene flow, and it has been argued that extensive genetic mixing among wildlife populations may increase the potential for viral epidemics [22] . Therefore, to characterize viral infection dynamics in wildlife populations, information on host population structure and connectivity is needed. Indeed, Plowright et al. [23] suggested that a large, weakly coupled asynchronous metapopulation structure might be necessary for population-level persistence of HeV with either acute ‘explosive’, or slow ‘smouldering’ epidemics resulting from spatial heterogeneity in population herd immunity. We recently demonstrated evidence of exposure to henipaviruses in the small, isolated population of E. helvum on the Gulf of Guinea island of Annobón, indicating that a metapopulation model may not be required for persistence of all henipaviruses [24] . The persistence of lyssaviruses in some temperate insectivorous bat species has been shown to depend on certain life history traits, including hibernation and birth pulses [25] , but persistence mechanisms in non-hibernating species, such as E. helvum , are unknown. 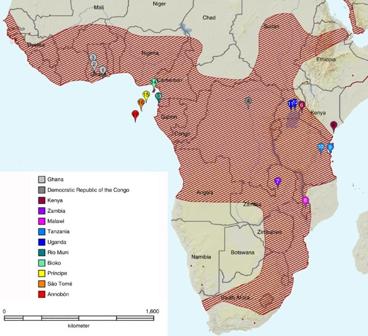Figure 1: Map showing location ofE. helvumsampling locations for genetic and serological analyses. Shading represents the distribution range ofE. helvum. Sampling locations are numbered as inSupplementary Data 1. Adapted with permission from Mickleburghet al.4 Figure 1: Map showing location of E. helvum sampling locations for genetic and serological analyses. Shading represents the distribution range of E. helvum . Sampling locations are numbered as in Supplementary Data 1 . Adapted with permission from Mickleburgh et al. [4] Full size image To determine the extent of genetic and epidemiological connectivity among E. helvum populations, and thus gain better understanding of viral transmission dynamics and zoonotic risk, here we combine genetic and serological analyses of populations across Africa. We use mitochondrial (mtDNA) and nuclear DNA analyses to characterize the range-wide metapopulation structure of E. helvum , and hypothesize that this would inform our understanding of viral dynamics across the population. Together with serological analyses, we assess the epidemiological consequences of this structure for the species’ ability to act as a reservoir host of the potentially zoonotic viruses, LBV and henipaviruses. Sampling Samples (including wing membrane biopsies, blood and urine) were obtained from 2,084 individual E. helvum bats across continental Africa and the Gulf of Guinea islands. In addition, pooled urine samples were collected from beneath some colonies. Details of sampling locations ( Fig. 1 and Supplementary Data 1 ) and sample sizes for genetic, serological and urine analyses ( Table 1 ) are provided. Table 1 E. helvum sample sizes and results for genetics and serological assays for individuals sampled from 12 populations. Full size table Microsatellite and mtDNA genetic analyses Overall, results from multiple analyses presented below showed that E. helvum forms a panmictic population across its continental range, with no evidence of isolation by distance (IBD) or structuring according to migratory routes. Bats on the offshore island of Bioko were found to be part of this panmictic population; however, the more isolated island populations in the Gulf of Guinea were genetically distinct from one another and from the continental population. 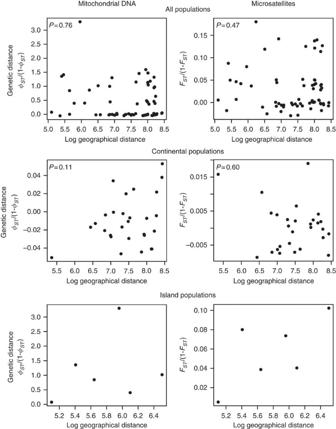Figure 2: Isolation by distance plots of pairwise population values for log geographic distance and genetic distance. Genetic distance is given by Slatkin’s linearizedφST(φST/(1-φST) for cytochromebmtDNA analyses (left column) or Slatkin’s linearizedFST(FST/(1−FST) for microsatellite analyses (right column). Note that the scales vary. Analyses were performed for allE. helvumpopulations (n=12), for continental populations only (n=8), or for island populations only (n=4). Statistical significance was assessed using a Mantel test andP-values are shown where sample size was sufficient to allow testing. Geographic distance is given in km. Of 114 unique cytochrome b ( cytb ) haplotypes identified from 544 individuals, 75% were singletons (only found in a single individual across all populations, Table 2 ). Haplotype diversity, molecular diversity, allelic richness and observed heterozygosity were all higher within continental with Bioko (CB) populations than in isolated island (iIS) populations. Nucleotide diversity was low across all populations, but particularly so in Príncipe and Annobón. Table 2 Molecular diversity of continental and island E. helvum populations. Full size table Structure among populations assessed by pairwise F ST (using microsatellite data) and φ ST (using mtDNA data) values gave similar results, with near-zero, non-significant values among CB populations, contrasting with larger, significant values between iIS and CB populations ( Supplementary Table S1 ). Each island population was also significantly differentiated from one another. 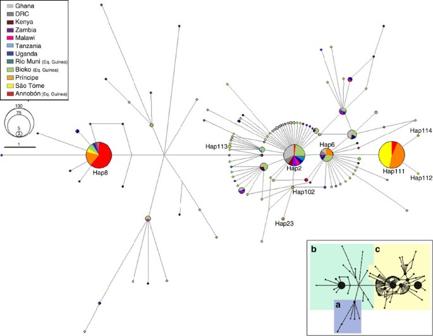Figure 3:Eidolon helvumcytochromebmedian joining haplotype network. No spatial clustering is present in continental African countries or within regions. Each circle represents a unique haplotype, and its size is proportional to its frequency. Lines represent base pair changes between two haplotypes, with the length proportional to the number of base pair changes. Main haplotypes and those containing island samples are labelled by name. Inset in the bottom right shows the relationship between the haplotype network and three clades identified in the Bayesian phylogeny. These results were supported by analysis of molecular variance (AMOVA), where maximal structure among groups (high F CT and φ CT values) and minimal structure among populations within groups (low F SC and φ SC ), were observed when populations were separated into three (CB, São Tomé with Príncipe (STP), Annobón) or four (CB, São Tomé, Príncipe, Annobón) groups ( Table 3 , analyses 7 and 8). IBD analyses detected no positive correlation between genetic distance (Slatkin’s linearized φ ST and F ST ) and log geographical distance in any mtDNA or microsatellite analyses ( Fig. 2 ). This finding was consistent when latitude was ignored and longitudinal distances were used in the analyses, accounting for presumed north–south migration routes of E. helvum [21] . Table 3 Structure of analyses and results of analysis of molecular variance Full size table Figure 2: Isolation by distance plots of pairwise population values for log geographic distance and genetic distance. Genetic distance is given by Slatkin’s linearized φ ST ( φ ST /(1- φ ST ) for cytochrome b mtDNA analyses (left column) or Slatkin’s linearized F ST ( F ST /(1− F ST ) for microsatellite analyses (right column). Note that the scales vary. Analyses were performed for all E. helvum populations ( n =12), for continental populations only ( n =8), or for island populations only ( n =4). Statistical significance was assessed using a Mantel test and P -values are shown where sample size was sufficient to allow testing. Geographic distance is given in km. Full size image A Bayesian phylogeny ( Supplementary Fig. S1 ) and median joining haplotype network ( Fig. 3 ) both recovered three main E. helvum clades. The star-like network was characterized by a few common haplotypes, surrounded by many haplotypes present in only 1–5 individuals. Thorough spatial mixing was evident, with the central haplotype (Hap2) being shared by 85 bats representing all CB populations plus a single bat from Annobón. Most bats from the isolated island (iIS) populations (253/272; 93%) were divided between two haplotypes at opposite ends of the network (Hap8, predominantly Annobón, and Hap111, predominantly STP; Supplementary Fig. S2 ). Figure 3: Eidolon helvum cytochrome b median joining haplotype network. No spatial clustering is present in continental African countries or within regions. Each circle represents a unique haplotype, and its size is proportional to its frequency. Lines represent base pair changes between two haplotypes, with the length proportional to the number of base pair changes. Main haplotypes and those containing island samples are labelled by name. Inset in the bottom right shows the relationship between the haplotype network and three clades identified in the Bayesian phylogeny. Full size image Consistent with these results, Bayesian clustering of individual genotypes revealed three clusters ( K =3) based on mean likelihood (log P (X|K) values ( Fig. 4 )), corresponding to populations from CB, STP and Annobón. With increasing values of K , the STP and Annobón clusters remained unchanged, and the CB cluster became increasingly subdivided into multiple clusters of approximately equal proportion ( Fig. 3 ), again indicative of a strong signature of a single panmictic CB population. Analyses run with CB or iIS samples as separate data sets did not reveal additional clusters. Using these three clusters as prior population information to identify potential migrants among clusters, STRUCTURE assignment tests (admixture analyses based on nuclear data), indicated that 19/502 individuals were ‘admixed’ (that is, had an assignment probability (p) to any one main cluster of 0.8>p>0.2). No bats were classified as recent (first generation) migrants ( Supplementary Table S2 ). 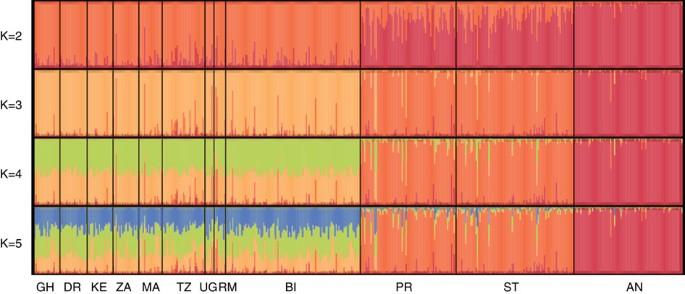Figure 4: Estimated population structure. Estimates from STRUCTURE analyses forK=2–5 based on microsatellite data from 502 individuals. Analyses run using the admixture setting identified three clusters corresponding to continental and Bioko populations (left), São Tomé and Príncipe (centre, orange) and Annobón (right, red). Each vertical line represents the proportional membership assignment of one individual to each ofKcoloured clusters. Black lines divide the plot into sampling locations. Ghana (GH), DRC (DR), Kenya (KE), Zambia (ZA), Malawi (MA), Tanzania (TZ), Uganda (UG), Rio Muni (RM), Bioko (BI), Príncipe (PR), São Tomé (ST), Annobón (AN). Figure 4: Estimated population structure. Estimates from STRUCTURE analyses for K =2–5 based on microsatellite data from 502 individuals. Analyses run using the admixture setting identified three clusters corresponding to continental and Bioko populations (left), São Tomé and Príncipe (centre, orange) and Annobón (right, red). Each vertical line represents the proportional membership assignment of one individual to each of K coloured clusters. Black lines divide the plot into sampling locations. Ghana (GH), DRC (DR), Kenya (KE), Zambia (ZA), Malawi (MA), Tanzania (TZ), Uganda (UG), Rio Muni (RM), Bioko (BI), Príncipe (PR), São Tomé (ST), Annobón (AN). Full size image Isolation-with-migration models and approximate Bayesian computation were unsuccessful in obtaining reliable estimates of gene flow between these islands, as a result of lack of convergence or unrealistically large estimates of effective population size, respectively. LBV serological analyses Using modified fluorescent antibody virus neutralization assays, neutralizing antibodies to LBV were detected in all continental and island locations ( Table 1 ), yet seroprevalences showed significant variation by geographical location. A strikingly low LBV seroprevalence relative to other locations was observed in the Annobón population ( χ 2 =66.5, P <0.001), but seroprevalences in Bioko, São Tomé and Príncipe were not significantly different from mainland populations. Excluding Annobón and populations with sample sizes that were insufficient to allow a reliable seroprevalence to be calculated (Malawi, Zambia and Uganda; n =12, 9 and 4, respectively), the mean LBV seroprevalence was 34% (95% CI: 32−37%) and the range of adult seroprevalences was 24–51% ( Supplementary Data 1 ). In the Annobón population, neutralizing antibodies to LBV were detected in 1 of 72 (1.4%, 0.0–7.5%) bats sampled in 2010 (ref. 24 ), and in 6 of 49 (14%, 7–27%) bats sampled in 2011. Henipavirus serological analyses Antibodies binding to NiV soluble G glycoproteins were detected using Luminex microsphere binding assays in all populations sampled ( Table 1 ). In contrast to the LBV results, henipavirus seroprevalences in all Gulf of Guinea islands (including Annobón) were similar to those in continental populations. Excluding populations with very small sample sizes, as above, the mean henipavirus seroprevalence was 42% (39−44%), with adult seroprevalences ranging from 29−60% ( Supplementary Data 1 ). Using virus neutralization tests (VNTs), a NiV seroprevalence of 5% (11/222, 3−9%) was detected in bats sampled from Tanzania and 1.7% (2/118, 0.5−6%) in bats from Annobón. For bats from Bioko, São Tomé and Príncipe, NiV VNTs were performed on a subset of the samples (those with binding assay median fluorescence intensities >750 ( n =49, 20 and 39, respectively)), of which 32, 50 and 51% were neutralizing, respectively. For both LBV and henipaviruses, no significant differences in seroprevalence were detected between males and females. Urine analyses Polymerase chain reactions (PCRs) performed on E. helvum urine samples from Tanzania, Uganda, Malawi, Zambia and Annobón detected paramyxovirus polymerase gene sequences in 3/23 extraction pools (from Ugandan and Tanzanian sampling sites, Table 1 ). These showed close relationships with sequences detected previously in E. helvum in Ghana [12] ( Fig. 5 ). One PCR-positive pooled sample from Tanzania comprises urine expressed directly from the bladders of six individual E. helvum , all of which were seronegative for henipaviruses using microsphere binding assays and VNTs. 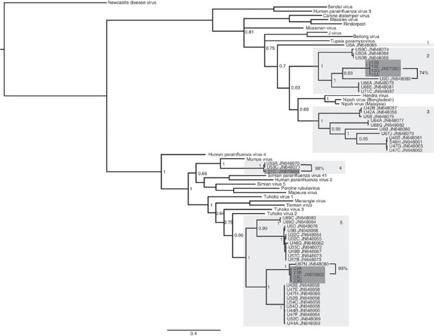Figure 5: Diversity of paramyxoviruses inEidolon helvumurine collected across multiple African sites detected usingParamyxovirinae-targeted PCR. Phylogenetic tree for a 531 bp segment of the polymerase gene of members of the subfamilyParamyxovirinae, including sequences generated in this study and publicly available paramyxovirus sequences (with GenBank accession numbers). Relevant posterior probability values are shown. Horizontal branches are drawn to a scale of nucleotide substitutions per site. Individual extraction pools IDs are followed by letters denoting the clone. Groups containing previously uncharacterized sequences that display a common phylogenetic origin supported by high posterior probability values (≥0.95) are highlighted by numbered light grey boxes. Within these boxes, sequences obtained from samples collected from Tanzania and Uganda are further highlighted by darker grey boxes. Pair wise nucleotide identities of the sequences from samples collected Tanzania and Uganda with their nearest phylogenetic relative are shown within the grey boxes. One PCR-positive Ugandan pooled sample (sample 23) contained paramyxoviral sequence with 95% nucleotide sequence identitywith sequences detected in Ghana that comprised part of a phylogenetically-distinct lineage of unclassified bat-derived viruses (group 5). Of the two PCR-positive Tanzanian samples, one contained paramyxoviral sequence related to mumps virus (sample 21) and shared 98% nucleotide identity with a Ghanaian sequence (group 2), and the other (sample 13) contained a sequence related to, but distinct from (74% nucleotide identity) sequences detected in Ghana (group 3). Figure 5: Diversity of paramyxoviruses in Eidolon helvum urine collected across multiple African sites detected using Paramyxovirinae -targeted PCR. Phylogenetic tree for a 531 bp segment of the polymerase gene of members of the subfamily Paramyxovirinae , including sequences generated in this study and publicly available paramyxovirus sequences (with GenBank accession numbers). Relevant posterior probability values are shown. Horizontal branches are drawn to a scale of nucleotide substitutions per site. Individual extraction pools IDs are followed by letters denoting the clone. Groups containing previously uncharacterized sequences that display a common phylogenetic origin supported by high posterior probability values (≥0.95) are highlighted by numbered light grey boxes. Within these boxes, sequences obtained from samples collected from Tanzania and Uganda are further highlighted by darker grey boxes. Pair wise nucleotide identities of the sequences from samples collected Tanzania and Uganda with their nearest phylogenetic relative are shown within the grey boxes. One PCR-positive Ugandan pooled sample (sample 23) contained paramyxoviral sequence with 95% nucleotide sequence identitywith sequences detected in Ghana that comprised part of a phylogenetically-distinct lineage of unclassified bat-derived viruses (group 5). Of the two PCR-positive Tanzanian samples, one contained paramyxoviral sequence related to mumps virus (sample 21) and shared 98% nucleotide identity with a Ghanaian sequence (group 2), and the other (sample 13) contained a sequence related to, but distinct from (74% nucleotide identity) sequences detected in Ghana (group 3). Full size image In this study, using data from both mtDNA and microsatellite markers, we demonstrate that the population of E. helvum is panmictic across its continental African range. An absence of IBD indicated that gene flow was no more likely to occur among neighbouring populations than distant populations of >4,500 km, making E. helvum the largest reported panmictic unit of any mammal, and one of the largest of any vertebrate, exceeded only by the bigeye tuna ( Thunnus obesus ; >8,000 km) [26] , [27] and the Kentish plover ( Chadadrius alexandrines ; >10,000 km) [28] . Even present day human populations retain genetic structure over such large distances [29] . In fact, the range of E. helvum extends further north and west of the sampling sites in this study, so additional sampling is required to assess whether panmixia extends across this range; a distance of >6,500 km. The hypothesis that greater genetic differentiation might exist across migratory pathways (on an east–west axis) than along migratory pathways (on a north–south axis) was not supported by our results, probably either because gene flow between distinct migratory populations homogenises allele frequencies, or because E. helvum migration is opportunistic and tracks changes in available food resources rather than following defined migratory routes. Included in the panmictic E. helvum population are bats on the near-shore island of Bioko in the Gulf of Guinea (which separated from the African continent ~7,000 years ago). Our results indicate that the 32 km stretch of ocean that separates Bioko from the continent is not a significant barrier to dispersal, as might be expected given that individuals are capable of covering such distances during foraging bouts [20] . In contrast to the panmictic continental and Bioko (CB) population, populations on the three more isolated Gulf of Guinea islands (São Tomé, Príncipe and Annobón) showed evidence of genetic isolation. This accords with the results from studies of other Gulf of Guinea island taxa, including other species of bat [30] , bird (for example, Melo et al. [31] ), and reptile (for example, Jesus et al. [32] ). Although E. helvum is a long-range migrant and has been observed as a vagrant on islands 570 km from the African coastline [33] , the strong genetic structure detected among the island and CB population clusters and the absence of genetic evidence (using assignment tests) of recent migrants between these clusters, indicate that dispersal between clusters (with successful mating) is likely to be rare: no first generation migrants were detected, although some individuals may have been second or third generation migrants. Additional support for population genetic results in this and other fruit bat species comes from genetic studies of external parasites and their pathogens [34] , [35] , including detection of congruence between population genetic structure of external parasites and their hosts. The Gulf of Guinea ocean channels are likely to have provided a barrier to initial colonization and inter-island dispersal. Also, we found that the smallest discrete population of E. helvum (on the island of Annobón) showed genetic divergence and is truly isolated. Our mtDNA and microsatellite results are consistent with those of a previous study that found that E. helvum on Annobón showed differences in morphological traits and allozyme frequencies compared with other islands [17] . However, while Juste et al. [17] also concluded that a lack of phenetic differentiation on Bioko, São Tomé and Príncipe suggested gene flow among the islands, our use of multiple nuclear and mtDNA markers, provides further insight. For example, while São Tomé shows greater connectivity with Príncipe (<150 km apart) than with either the CB or the Annobón populations (which lie >220 km away), the distance separating these two populations is still a substantial barrier to inter-island gene flow, as shown by significant pairwise φ ST and F ST values. As São Tomé and Príncipe are within the same cluster, it is not possible to identify migrants between these two islands using assignment tests. Other genetic methods to estimate gene flow and demographic history between multiple populations, including isolation-with-migration models and approximate Bayesian computation, were unsuccessful in obtaining reliable and credible estimates of gene flow between these islands, suggesting that even for our substantial data sets, modelling of low rates of gene flow using current techniques and assumptions is not robust. Although genetic analyses cannot replace direct studies on individual bat movements and demographic connectivity, they can contribute to a broader perspective upon which epidemiological studies on transmission and maintenance of viruses among and within populations can be based [36] . The strong genetic clustering observed here makes it likely that the separation of E. helvum into three distinct genetic population clusters (CB, STP and AN) is echoed as at least three epidemiologically distinct populations. A freely mixing, panmictic continental population would likely facilitate viral transmission among E. helvum colonies across this range. Our serology results are consistent with this, with henipavirus and LBV antibodies being detected across all continental sampling sites at seroprevalences similar to those previously observed for henipaviruses in Ghana [3] and for LBV in Ghana, Kenya and Nigeria [5] , [6] , [7] , [37] . Further support for the conclusion that distant continental populations may belong to a single epidemiological unit was provided by high nucleotide sequence identities between paramyxoviral sequences detected in E. helvum urine samples from Uganda and Tanzania and those already reported from Ghana [12] . In that study and others [13] , [38] , a diverse range of paramyxovirus sequences, including henipavirus-like sequences, were detected within single E. helvum populations. Further sampling efforts to enable exploration of viral sequence diversity across all the sites studied here would help determine whether different virus variants are maintained by each of these distinct epidemiological units and whether viral diversity may have a role in within-population viral persistence. Additional data are required to fully understand how virus variants are maintained within E. helvum populations. Although genetic differentiation and isolation of E. helvum in the STP cluster was expected to be reflected epidemiologically, perhaps with an absence of antibodies on these islands due to restricted population sizes, we found that seroprevalences to both viruses were comparable with those on the mainland. These data suggest that: population sizes on each island are sufficient to maintain LBV and henipaviruses and are above the CCS required for persistence (although this concept requires further theoretical exploration for animal populations where birth rates, and hence population sizes, are highly seasonal); sufficient movement may occur between the two islands to maintain a larger epidemiologically connected population; alternative hosts may be involved; or our original assumptions on transmission and persistence may need re-examination (see below). The use of satellite telemetry has been enlightening in other fruit bat species [39] , [40] and would be required to definitively assess movement patterns of bats on these two islands. However, dispersal between São, Tomé and Príncipe was suggested by our observation of a single asynchronous birth on Príncipe in the absence of other pregnant or lactating females, but which was contemporaneous with the presence of neonates on São, Tomé. The asynchronous Príncipe birth is highly unusual for a species, which employs delayed implantation to facilitate a highly synchronized birth pulse. If the two populations are connected via dispersal, the asynchrony in reproductive seasons between São Tomé and Príncipe could facilitate viral persistence by staggered introduction of susceptible individuals, via birth, into the population. Finally, LBV has been detected in bats of several species in Africa, with ranges overlapping that of E. helvum [2] , but the role that interspecies transmission has in the maintenance of LBV in its host populations remains a gap in our knowledge. Of all these species, only Rousettus aegyptiacus , the Egyptian fruit bat, is present on São, Tomé and Príncipe. This is a cave-roosting species, and mixed colonies with E. helvum are unlikely, although these two species might mix at feeding sites. LBV has been isolated from R. aegyptiacus on two occasions (as reviewed in Kuzmin et al. [41] ), and seroprevalence levels comparable with those reported in E. helvum were detected in Kenya [6] . On São, Tomé and Príncipe, R. aegyptiacus , or indeed other species, may facilitate the persistence of LBV in E. helvum . Although findings from the CB and STP populations could be consistent with a metapopulation model of persistence, as proposed for HeV in Australia [23] and NiV in Malaysia [42] , our results from Annobón indicate that this appears unnecessary for the persistence of henipaviruses or LBV in E. helvum . On Annobón, E. helvum is the only bat species confirmed to be currently present and has a population size of only ~2,500 (ref. 24 ). Surprisingly, and in contrast to findings in other, less-isolated island systems [42] , the henipavirus seroprevalence in the Annobón E. helvum population was within the range of that observed in both the CB and the STP populations. Conversely, the Annobón LBV seroprevalence was much lower than in other populations. Although evidence of infection with lyssaviruses has been reported in other island bat species (for example, refs 43 , 44 ), the bat populations in those studies were either much larger, within flight distance of continental bat populations, and/or hosted multiple sympatric bat species. In Annobón, all LBV seropositive individuals were adult, and further longitudinal studies are required to determine whether LBV is persistently maintained on this island (that is, the population size is greater than the CCS), or whether these findings represent a single epidemic wave subsequent to introduction of the virus from another population. Unfortunately, deriving a quantitative estimate for the CCS is problematic, particularly for virus-host systems where little information is available regarding host demographics, virus transmission mechanisms and within-host immune responses [45] . For both LBV and henipaviruses, important areas of future study include viral diversity and phylogeography, within-host persistence and immunity, incubation periods and frequency- versus density-dependent transmission. Multiple henipavirus-like sequences have been previously reported in E. helvum [11] , [12] , [13] . In the absence of isolation or full genomic characterization, it cannot be definitely confirmed whether these sequences represent true henipaviruses. However, a phylogenetic analysis undertaken here, incorporating the most recently isolated henipavirus (CedPV in Australia) and sequence fragments from bat paramyxoviruses worldwide ( Fig. 6 ) demonstrate that two virus sequences from E. helvum in Gabon [13] fall within the clade of currently identified henipaviruses. These sequences therefore likely represent true African henipaviruses. 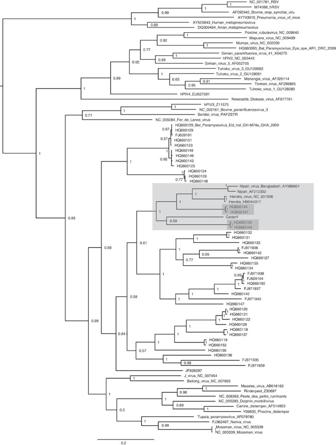Figure 6: Henipavirus phylogenetic relationships. Phylogeny based on a 559 bp segment of the polymerase gene incorporating fragments known Paramyxovirinae and fragments from Drexleret al.13The clade containing known henipaviruses (Hendra virus (HeV), Nipah Virus (NiV) and Cedar virus (CedPV)) is highlighted in pale grey. Sequence fragments from viruses detected inE. helvumwithin this clade are further highlighted by dark grey boxes. Posterior probability values are shown and the bar represents 0.2 expected nucleotide substitutions per site. GenBank accession numbers are shown. Figure 6: Henipavirus phylogenetic relationships. Phylogeny based on a 559 bp segment of the polymerase gene incorporating fragments known Paramyxovirinae and fragments from Drexler et al . [13] The clade containing known henipaviruses (Hendra virus (HeV), Nipah Virus (NiV) and Cedar virus (CedPV)) is highlighted in pale grey. Sequence fragments from viruses detected in E. helvum within this clade are further highlighted by dark grey boxes. Posterior probability values are shown and the bar represents 0.2 expected nucleotide substitutions per site. GenBank accession numbers are shown. Full size image This study took a multidisciplinary approach, combining ecological, genetic and serological studies, to explore the ways in which the structure, dynamics and connectivity of E. helvum populations across Africa affects the viral transmission dynamics within them. These critical population-level processes are expected to be important in determining viral persistence within populations, and yet, although the three genetically distinct populations identified here are also highly likely to be separated epidemiologically, each of these population clusters is capable of maintaining henipaviruses and LBV, apparently without the need for a metapopulation model of persistence via migration and reintroduction. The findings presented here have potentially important implications for public health. The large population sizes of E. helvum , its tendency to roost and feed in close proximity to human populations, its extensive distribution across Africa and its frequent harvesting for bushmeat, present numerous opportunities for the exposure of people to excreta, tissues and body fluids from these bats. The widespread presence of potentially zoonotic viruses in this species across Africa might therefore be of significant public health concern. Despite the possibility for undiagnosed spillover, the lack of detection makes it unlikely that pathogenic henipaviruses from E. helvum are regularly crossing the species barrier and undergoing significant sustained transmission in humans at this point in time. Spillover of NiV into pig populations in Malaysia may have occurred at least once prior to the detection of a major outbreak [46] , and therefore, detection of henipavirus antibodies in pigs in Ghana [47] warrants further study. Although no human cases of LBV infection have been reported, this virus causes clinical rabies in other mammalian hosts [2] , and may not be detected as a cause of human rabies unless specific molecular-based LBV assays are performed. Changes in bat–human interactions and bat–domestic animal interactions are hypothesized to be a catalyst for the zoonotic spillover of novel viruses from wildlife. Stressors, such as habitat loss, land-use change and increasing bat–human interactions may precipitate viral spillover from bats to other species [23] . Understanding viral persistence and the potential for spillover in African bat populations in the face of extensive hunting, logging and human population growth is of central importance for both public health and conservation, especially as these processes can be expected to increase over time. Sampling All fieldwork was undertaken under permits granted by national and local authorities, with ethical approval from the Zoological Society of London Ethics Committee (project reference WLE/0489). Personal protective equipment (long clothing, facemasks, eye protection and gloves) was worn during sample collection. Sampling was conducted in geographically widespread E. helvum populations along longitudinal and latitudinal axes across the species’ range ( Fig. 1 , Supplementary Data 1 ). In São Tomé, bats were obtained in collaboration with local hunters, who hunted at roost sites during the day or feeding sites at night. Elsewhere, bats were captured at the roost with mist nets (6–18 m; 38 mm) as they departed the roost site at dusk, or returned at dawn. Female reproductive status was assigned as non-reproductive, pregnant or lactating, assessed visually or via abdominal palpation. Age was assessed by morphological characteristics and all individuals could be allocated into one of four age classes: neonate (<2 months), juvenile (J; 2—<6 months), sexually immature (SI; 6—<24 months) or adult (A; ≥24 months). For a subset of samples, the timing of sampling allowed further classification of SI individuals into 6-month age groups SI.1, SI.2 and SI.3 (6<12, 12—<18, 18—<24 months, respectively). Genetic and blood samples were collected under manual restraint. Wing membrane biopsies (4 mm) were placed into 70% alcohol. Up to 1 ml blood was collected from the propatagial vein using a citrated 1-ml syringe and placed into a plain 1.5 ml Eppendorf tube. Pooled urine samples (up to 500 μl) were collected by pipette from plastic sheeting placed under E. helvum colonies in Tanzania and Uganda at dawn [12] , or directly from individual bats (in Tanzania, Malawi, Zambia and Annobón), and frozen at −80 °C without preservative. ‘Populations’ were initially defined arbitrarily based on national borders related to roost location. Molecular methods Genomic DNA was extracted from E. helvum tissues using DNeasy Blood and Tissue Kits (Qiagen, Crawley, West Sussex, UK) and was supplied for one E. dupreanum bat from Madagascar by the Institut Pasteur de Madagascar. Multiplexed genotyping was performed using 18 loci in six multiplexed reactions (TSY, FWB, MNQX, AgPK, AcAfAi, AdAh) using a Type-it Multiplex PCR Master Mix (Qiagen). From 20 E. helvum loci developed in a previous study [48] , Loci E and Ae were discarded due to difficulty in scoring or high error rates and data pertaining to locus Ag were re-binned and re-scored, correcting earlier issues with allelic dropout. Positive and negative controls were included on each plate. Amplification of mtDNA cytb gene fragments from continental samples used generic primers L14722 (5′-CGA AGC TTG ATA TGA AAA ACC ATC GTT G-3′) [49] and H15149 (5′- AAA CTG CAG CCC CTC AGA ATG ATA TTT GTC CTC A-3′) [50] in 20 μl reactions, containing 0.1–1 ng template DNA, 0.2 μM of each primer, 0.25 mM of each dNTP, 1.5 mM MgCl 2 , 0.25 μl of Taq polymerase (Invitrogen), and 0.2 μl 10 × reaction buffer and with the following conditions: 5 min at 94 °C; 40 cycles of 1 min at 93 °C, 1 min at 54 °C and 2 min at 72 °C; then 7 min at 72 °C. Although these generic primers were adequate with continental samples (8% PCR failure), amplification from isolated Gulf of Guinea island samples was less successful (48% PCR failure). Shortened primers (EhM2814 (5′-GCT TGA TAT GAA AAA CCA TCG TTG-3′) and EhM2815 (5′-CAG CCC CTC AGA ATG ATA TTT GT-3′) resulted in successful amplification when using Microzone MegaMix-Gold reagent (Microzone UK). PCRs were performed in 20 μl reactions, containing 2 ng template DNA, 0.25 μM of each primer and 10 μl MegaMix-Gold, using the following conditions: 5 min at 95 °C; 33 cycles of 30 s at 95 °C, 30 s at 53 °C and 45 s at 72 °C. PCR products were sequenced in both directions, aligned, manually checked and trimmed to 397 bp. No sequence differences were detected in 38 samples sequenced using both primer pairs, so data were combined. RNA was extracted from urine samples using the MagMAX viral RNA isolation kit (Life Technologies, Paisley, UK), and the presence of paramyxovirus polymerase gene RNA was tested for using two heminested RT–PCRs ( PAR-F2 : 5′-GTT GCT TCA ATG GTT CAR GGN GAY AA-3′, PAR-R : 5′-GCT GAA GTT ACI GGI TCI CCD ATR TTN C-3′) [12] , [51] . Genetic data analyses After removing non-independent samples (known or suspected offspring of other individuals within the data set), cytb analyses and microsatellite analyses (at 17 loci) were performed on data from 544 and 502 individuals, respectively ( Table 1 ). Abbreviations for population groupings used in analyses are CT (all continental populations), CB (all continental populations plus Bioko), IS (all four island populations), iIS (three isolated island populations (São Tomé, Príncipe and Annobón)) and STP (São Tomé and Príncipe) ( Supplementary Fig. S3 ). The statistical power of the microsatellite and mtDNA data sets to reject a null hypothesis of genetic homogeneity was assessed using the software POWSIM [52] . Values from the empirical data sets (number of populations, population sample sizes, number of loci and allele frequencies) were used to simulate 1,000 random sets of 12 subpopulations with expected F ST values of 0.001−0.01. As mtDNA is haploid, the sample size was halved for mtDNA analyses. Power calculations indicated that the inability to detect population structure among CB populations was not because of insufficient power within the data set, and the estimated probability of falsely detecting significant differentiation was in line with the typically accepted 0.05 cutoff. Analyses were therefore continued as described below. For microsatellite data, departures from Hardy–Weinberg equilibrium (HWE) and the presence of linkage disequilibrium among loci were assessed using FSTAT v2.9 (ref. 53 ) and GENEPOP v4.0.10 (ref. 54 ), respectively. Significance levels were adjusted for multiple testing using the false discovery rate method. Genetic diversity for each population and region was assessed by calculating observed heterozygosity ( H O ), expected heterozygosity ( H E ), and average allelic richness ( R S ) in FSTAT. Population structure was assessed by calculating pairwise F ST values between populations and by AMOVA, as implemented in the software ARLEQUIN v3.5 (ref. 55 ). Significance levels were obtained with 10,000 permutations. Data were tested for the presence of IBD by regressing natural logarithm-transformed geographical distances between sampling sites (in km) against Slatkin’s linearized F ST ( F ST /(1- F ST )). Statistical significance was assessed using a Mantel test with 10,000 permutations in ARLEQUIN. Bayesian clustering analyses were performed 20 times for each value of K ( K =1–13, representing the number of populations) for 1.5 × 10 6 iterations with 500,000 burn-in steps using the admixture model with correlated allele frequencies in STRUCTURE [56] . Analyses were repeated for separate continental and island data sets. Symmetric similarity coefficients were used to assess consistency among replicate runs for each value of K using the Greedy algorithm of CLUMPP v1.1 (ref. 57 ), and only runs with symmetric similarity coefficients >0.8 were included in further analyses. Individual membership coefficients from replicate runs were visualized graphically using the software DISTRUCT v1.1 (ref. 58 ). To ensure that some loci not in HWE in the Bioko populations (see results) were not affecting clustering from this population, analyses were repeated separately with data from loci in or out of HWE in Bioko. No difference was seen in the results, and therefore remaining analyses were run with 16 loci. Assignment tests were performed in STRUCTURE and admixture was assessed using the USEPOPINFO option, using the clustering partition with the optimal mean log likelihood value as prior population information. Based on their assignment probability, P , individuals were considered non-migrant ( P >0.8), admixed (0.2> P >0.8) or a recent migrant ( P <0.2) [59] . STRUCTURE and CLUMPP analyses were performed using the CamGrid distributed computing resource. Comparable analyses were performed using spatially explicit methods; however, the results were consistent and are not presented here. For mtDNA, in addition to AMOVA and IBD analyses, descriptive parameters of genetic diversity were calculated in the software DnaSP v5.10 (ref. 60 ). Rarefaction down to the minimum sample size was used to calculate haplotypic richness (a measure of diversity standardized across population sample sizes) using the software RAREFAC [61] . Pairwise φ ST values were calculated in ARLEQUIN and significance values were adjusted for multiple comparisons using the false discovery rate method. Median joining networks (MJNs) were constructed in the software NETWORK v4.6 (ref. 62 ). For comparison, statistical parsimony networks were constructed using TCS [63] , with a 95% parsimony connection limit; however, the results were consistent and are not presented here. A phylogeny of unique cytb haplotypes was reconstructed by Bayesian inference in MRBAYES v3.1.2 (ref. 64 ), using the E. dupreanum cytb sequence as an outgroup (which was found to be 91% (360/397 bp) identical to the consensus E. helvum cytb sequence). The most appropriate substitution model (GTR+I) was selected using PAUP* v4.0b10 (ref. 65 ) and MODELTEST v3.7 (ref. 66 ). MRBAYES was run with four simultaneous chains, sampled every 100 generations and the first 25% of trees were discarded as burn-in. Generations were added until the s.d. of split frequencies was below 0.015 (10 × 10 6 generations). The relative contributions of isolation and gene flow (migration) on observed levels of population divergence were estimated using an isolation-with-migration model in IMa2 (ref. 67 ). Once priors had been optimized, analyses were run until stationarity was reached, which took ~2–3 months and 1.7–46 million steps, depending on sample size, before genealogy sampling commenced. Genealogy information was saved every 100 steps, and sampling was continued until ~100,000 genealogies were available for each pairwise comparison (~1 month, depending on sample size). Eight competing colonization scenarios were explored by analysing microsatellite and mtDNA data using approximate Bayesian computation methods in the software DIYABC v 1.0 (ref. 68 ). Eight different colonization scenarios were considered. To construct a phylogenetic analysis of known henipaviruses and henipavirus-like viruses globally and other known Paramyxovirinae, sequences of a 559 bp segment of the polymerase gene were obtained from GenBank ( Supplementary Table S3 ). Phylogenetic trees from these sequences and of viral sequences from urine samples analysed in this study were constructed using MRBAYES under the GTR+I+G model. Serological analyses The number of samples analysed using various serological assays for HeV, NiV and LBV is shown in Table 1 . Antibodies against LBV (LBV.NIG56-RV1) were detected using a modified fluorescent antibody virus neutralization assay [37] , using the LBVNig56 isolate. Samples were tested in duplicate using threefold serial dilutions and titres corresponding to 100% neutralization of virus input are reported as IC100 endpoint reciprocal dilutions and were considered positive at >1:9. Antibodies against henipaviruses (HeV and NiV) were detected using Luminex multiplexed microsphere binding assays and VNTs using purified recombinant expressed henipavirus soluble G glycoproteins [69] , which were conjugated to internally coloured and distinguishable microspheres, allowing multiplexing. Antibody binding to each microsphere was detected after conjugation of bound antibodies with biotinylated protein A and fluorescent streptavidin-R-phycoerythrin. Binding results are given as MFI values of at least 100 microspheres for each virus type, and an MFI >500 was considered positive [70] . Alternative, lower cutoffs were also considered based on results from mixture model analyses [70] . These resulted in higher seroprevalences, but no overall change in patterns to the higher, more conservative, cutoff presented here. In VNTs, samples exhibiting virus neutralization at dilutions of ≥1:10 were considered positive. Stronger results were consistently observed in NiV binding assays and VNTs [24] , so only NiV results are reported here. χ 2 tests were used to detect significant ( P <0.05) variations in seroprevalences. Accession numbers: All sequences reported in this study have been deposited in the GenBank nucleotide database under accession numbers KC164869 to KC164982 ( Eidolon helvum cytochrome b mtDNA) and JX870901 to JX870903 (paramyxovirus polymerase gene sequences from E. helvum urine). How to cite this article: Peel, A. J. et al. Continent-wide panmixia of an African fruit bat facilitates transmission of potentially zoonotic viruses. Nat. Commun. 4:2770 doi: 10.1038/ncomms3770 (2013).